Controlled stripes of ultrafine ferroelectric domains In the pursuit of ferroic-based (nano)electronics, it is essential to minutely control domain patterns and domain switching. The ability to control domain width, orientation and position is a prerequisite for circuitry based on fine domains. Here, we develop the underlying theory towards growth of ultra-fine domain patterns, substantiate the theory by numerical modelling of practical situations and implement the gained understanding using the most widely applied ferroelectric, Pb(Zr,Ti)O 3 , demonstrating controlled stripes of 10 nm wide domains that extend in one direction along tens of micrometres. The observed electrical conductivity along these thin domains embedded in the otherwise insulating film confirms their potential for electronic applications. Ferroics such as ferromagnets and ferroelectrics are materials that undergo a ferroic transition between phases having point group/sub-group relationship [1] . This implies multistability below the ferroic phase transition and results usually in switchability of the order parameter under the conjugated external stimulus: magnetic field for ferromagnets and electric field for ferroelectrics. Owing to their multistability, ferroics are considered attractive for memories in addition to their wide-spread other applications in electromechanics and electronics. Domains are regions in the ferroic in which the order parameter (polarization, magnetization, and so on) is oriented in one of the symmetry permitted directions. Domain walls, the interface between adjacent domains, have the width of 10–100 nm in ferromagnets and 1–10 nm in ferroelectrics. Their properties can be different from those of the domains themselves [2] , [3] , [4] . Electronic conductivity was discovered at ferroelectric domain walls in BiFeO 3 (ref. 5 ). Charged walls in the common ferroelectric BaTiO 3 showed electron-gas-like conductivity, whereas the individual domains remained excellent insulators [6] . Large photovoltages were generated by domain walls in BiFeO 3 (ref. 7 ). The evidence of exploitable electrical properties of ferroic walls inspires research towards domain-wall nanoelectronics [8] , [9] . The possibility to create controlled arrays of domains having width comparable to that of domain walls has been rarely discussed and the properties of such entities are not known. Here, a first challenge is the creation of ordered fine domain-stripes. For very thin films, the existence of 180° stripe domains was evidenced [10] . They were shown not to be straight but instead to form a meandering pattern [11] . Here we focus on the creation of stripe arrays of ferroelastic, non-180°, ultrafine domains during film growth. Such structures, having ferroelastic domain walls, are more robust compared with those purely ferroelectric, which can be sensitive to the screening conditions. Combining this with a simple post-growth writing of purely ferroelectric (180°) domains, for example, using a cantilever tip, will result in complex patterns, where the different types of domain/domain walls will be the building blocks of the electronic circuit. Previous experimental work centred on domain walls in BiFeO 3 films [7] , [12] , [13] , [14] , [15] , where domain stripes are typically wide, ~100 nm, and width control is neither attempted nor discussed. In our work, we aim to control domain patterns at an order of magnitude finer scale, in which domain walls of finite width occupy substantial volume fraction (>10%) of the domain region. We use the impositions because of ferroelasticity and ferroelectricity to control ferroelectric/ferroelastic domain patterns. The existence of an a/c domain structure was observed before in PbTiO 3 on DyScO 3 substrates [16] , and the domain width of an anisotropic a/c domain pattern was compared with existing theory [17] . However, no direct evidence for the origin of the anisotropy was given, which would allow controlling the final pattern. We develop theory for the description of ultrafine ferroelastic domains and their sparse arrays, which was not covered by existing theories [18] , [19] , [20] , [21] , [22] , [23] . We address with this theory and show experimentally the making of stripe arrays of 7–10 nm wide domains. In this particular case, the domain region itself may display unique intrinsic properties because of large inhomogeneous strains, as discussed later. We demonstrate more complex patterns made through growth and post-growth manipulation of the films. Finally, electrical conductivity is found along these ultra-narrow domains of the otherwise insulating Pb(Zr,Ti)O 3 (PZT). Towards ultrafine stripes of ferroelectric domains We address the energetics of a/c domain patterns for tetragonal (001) film (the common ferroic species ) deposited onto pseudo-cubic substrate having lattice parameters closely matching the a-lattice constant of the ferroelectric. It is in this situation that formation of ultra-thin ferroelectric/ferroelastic domains with a very small a-domain fraction is expected having a period larger than the film thickness. For films with bottom electrodes, which are of interest here, the electrostatic contribution to the energy balance may be neglected as long as patterns with intersecting domain inclusions are not addressed. An important parameter controlling the features of a/c patterns in ferroelectric films is the formation energy of an individual a-domain inclusion in the c-monovariant [24] . This energy (per unit length of the inclusion) is the sum of the variation of elastic energy and self-energy of two inclined domain walls parallel to each other, where h and λ are film thickness and self-energy per unit area of the wall, respectively. We extend the results for square lattice termination [25] to the general case of pseudo-cubic substrates. For the present case, where we aim for a-domain width, w d , appreciably smaller than film thickness, an approximate relationship for the formation energy reads ( Supplementary Equation 18 in the Supplementary Discussion , derived using Supplementary Equations 1–17 and Supplementary Figs 1–3 ) where ξ= w d / h <1/2, α =( c–a )/ a is the tetragonality factor, a and c are the lattice constants of the bulk ferroelectric, and E and ν are Young modulus and Poisson ratio, respectively, taken identical for both film and substrate. For square substrate termination with in-plane lattice constant a s ( c>a s >a ) , γ = γ 0 =(1– ν ) ϕ , where ϕ =( a s –a )/( c–a ) is the relative coherency strain. Equation (1) yields equal formation energies of a-domain for the two possible orientations ( Fig. 1a ). 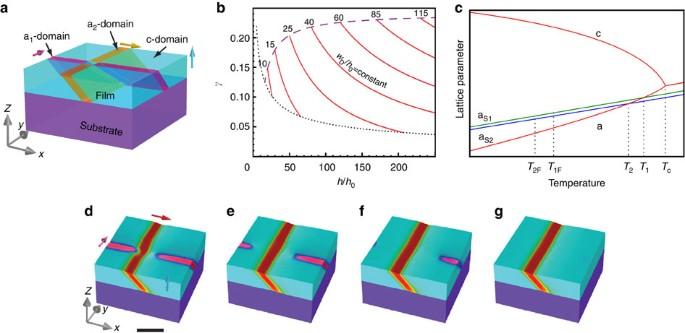Figure 1: Theoretical analysis of heteroepitaxial system. Tetragonal ferroelectric grown on orthorhombic (pseudo-cubic) substrate. (a) Illustration of allowed domain orientations. The polarization direction (indicated by coloured arrows) in the tetragonal films is along thecaxis of its unit cell. a-Domains have oneaaxis of the unit cell perpendicular to the surface of the film and the polar axis lying in the plane of the film, parallel to the []Sor [001]Sorientation of the pseudo-cubic orthorhombic substrate (orthorhombic notation of Miller indices, the subscript s denotes the substrate). (b) Stripe domain geometry in terms of the film thicknesshand the coherency factorγ. The solid curves (red—online) correspond to a constant width of the a-domainswd; the numbers at the curves give the widthwdmeasured in units ofh0given by equation (5) of the main text. The upper dashed curve shows the limit of the applicability of the approximation used in the calculation,wd/h<1/2. The area below the dotted curve corresponds to the c-monovariant. (c) Schematic of temperature dependence of lattice constants of the tetragonal film clamped to the anisotropic substrate:aandc—lattice parameters of the film,as1andas2—long and short axis of the anisotropic substrate.TCdepicts the Curie temperature, shifted by the clamping. At temperaturesT1andT2, the misfit strains along the long and short pseudo-cubic axes of the substrate change the sign, respectively. At temperaturesT1FandT2F, the formation of a-domains (in the c-domain matrix) normal to the long and short pseudo-cubic axes (easy and hard domains) becomes energetically favourable. (d) Phase-field calculated cross-hatched pattern. The model assumes periodic boundary conditions (see Methods). (d–g) Illustrate meta-stability of a-domain crossing. A small variation of simulation parameters like temperature, film thickness or domain wall energy (used in this case) dictates whether the a-domain crossing is stabilized or not. Here the increase of domain wall energy leads to disappearance of one type of a-domains. The scale bar is 50 nm. Figure 1: Theoretical analysis of heteroepitaxial system. Tetragonal ferroelectric grown on orthorhombic (pseudo-cubic) substrate. ( a ) Illustration of allowed domain orientations. The polarization direction (indicated by coloured arrows) in the tetragonal films is along the c axis of its unit cell. a-Domains have one a axis of the unit cell perpendicular to the surface of the film and the polar axis lying in the plane of the film, parallel to the [ ] S or [001] S orientation of the pseudo-cubic orthorhombic substrate (orthorhombic notation of Miller indices, the subscript s denotes the substrate). ( b ) Stripe domain geometry in terms of the film thickness h and the coherency factor γ . The solid curves (red—online) correspond to a constant width of the a-domains w d ; the numbers at the curves give the width w d measured in units of h 0 given by equation (5) of the main text. The upper dashed curve shows the limit of the applicability of the approximation used in the calculation, w d / h <1/2. The area below the dotted curve corresponds to the c-monovariant. ( c ) Schematic of temperature dependence of lattice constants of the tetragonal film clamped to the anisotropic substrate: a and c —lattice parameters of the film, a s1 and a s2 —long and short axis of the anisotropic substrate. T C depicts the Curie temperature, shifted by the clamping. At temperatures T 1 and T 2 , the misfit strains along the long and short pseudo-cubic axes of the substrate change the sign, respectively. At temperatures T 1F and T 2F , the formation of a-domains (in the c-domain matrix) normal to the long and short pseudo-cubic axes (easy and hard domains) becomes energetically favourable. ( d ) Phase-field calculated cross-hatched pattern. The model assumes periodic boundary conditions (see Methods). ( d – g ) Illustrate meta-stability of a-domain crossing. A small variation of simulation parameters like temperature, film thickness or domain wall energy (used in this case) dictates whether the a-domain crossing is stabilized or not. Here the increase of domain wall energy leads to disappearance of one type of a-domains. The scale bar is 50 nm. Full size image For pseudo-cubic substrates having different in-plane lattice constants a s1 and a s2 , c>a s1 >a s2 >a , the a-domain inclusion energy normal to the a s1 axis of the substrate is described with equation (1), where γ = γ 1 ≡ ϕ 1 + vϕ 2 , ϕ 1 =( a s1 – a )/( c – a ) and ϕ 2 =( a s2 – a )/( c – a ). For the inclusion energy normal to a s2 , (1) is used with γ = γ 2 ≡ ϕ 2 + vϕ 1 . Thus, the energetics of a-domain formation is essentially controlled by the γ parameter, which characterizes the film’s stress state (hereafter called coherency factor). Minimization of equation (1) with respect to ξ gives the relationship between γ and the equilibrium width of a-domains: The corresponding energy-reduction due to stress release is: This energy reduction is the driving force for domain formation. Once |Δ F | becomes larger than the energy paid for domain wall formation, , a-domain can appear. This is possible once the film thickness exceeds a critical value h cr (ref. 26 ) corresponding to the condition (more precisely ), yielding where h 0 is the length scale introduced by Roytburd [27] for the description of a/c patterns in ferroelectric thin films. For typical perovskites like PZT, h 0 is of the order of 1 nm (ref. 1 ). The above treatment describes adequately a-domain formation when the distance between domains is large enough to neglect elastic coupling between them. Otherwise, this coupling should be taken into account, as shown below. Our calculations ( Supplementary Equations 40 and 41 , derived using Supplementary Equations 19–39 and Supplementary Figs 4–7 ) give a generalized form of equation (2), for the case of one-dimensional periodic lamellar pattern of a-domains having period l >> h : The calculations for the period yield Thus, the geometrical parameters of the stripe pattern, width w d =h ξ and period l of a-domains are controlled by film thickness h and two material-related parameters: the length scale h 0 , which is a property of the ferroelectric, and coherency factor γ , which characterizes the film’s stress state. To tailor a-domain width for a given material, one can control film thickness and coherency factor based on the diagram ( Fig. 1b ) derived using equations (6) and (7). Note that, in view of equations (6) and (7), in the limit of small films’ thickness, approaching the critical value of h cr =0.16 h o γ −9/4 , the structure period and a-domain width scale as and w d ∝ h , respectively, having nothing in common with the Kittel-type law, often used for the interpretation for the domain data for ferroelectric films. Applying the above analysis to equilibrium stripe a/c domain patterns for in-plane square-lattice substrate-termination suggests that formation of a-domains in both possible orientations is equally probable and cross-hatched domain patterns are expected. However, in a pseudo-cubic substrate having different in-plane (pseudo-cubic) lattice constants, the anisotropy of the substrate’s in-plane lattice constants can influence whether stripe or cross-hatched a/c pattern will form at the transition from cubic to tetragonal phase, even if isotropic elastic moduli are assumed. Competition between stripe and cross-hatched patterns The problem of the competition between the stipe and cross-hatched domain patterns has been theoretically addressed in the past [28] , [29] , [30] . However, only in equilibrium situations with dense patterns or with linear coupling between the order parameter and strain have been under the consideration so that the results obtained cannot be directly applied to our system exhibiting a sparse pattern of narrow domains. In this section, we will theoretically treat the situation where a sparse pattern of narrow a-domains forms on a substrate with a very weak anisotropy of in-plane lattice constants. In view of domain wall pinning, equilibrium theory cannot be directly applied in the case where energies of two possible states (formation of stripes in two perpendicular directions) are only slightly different. Below we implemented an element of kinetics by tracing the sample on its cooling from the high-temperature phase. Consider temperature dependences of the ferroelectric bulk lattice constants and the in-plane lattice constants of the substrate a s1 and a s2 ( Fig. 1c ) and a small substrate anisotropy a s1 –a s2 ≪ c–a . Upon cooling and just below the ferroelectric transition, the film is under compressive stress in both directions, thus the c-monovariant is energetically preferred. On further cooling, the strain changes to tensile, first along the longer a s1 axis, at temperature T 1 ( Fig. 1c ). Just below T 1 , the formation of a-domains normal to the a s1 axis (hereafter such domains are called easy domains) would lead to a certain stress release. However, easy domain formation is energetically favourable only if the elastic energy gain ( cf . equation (3) ) substantially compensates the energy penalty due to walls self-energy, that is, The corresponding critical temperature T 1F ( Fig. 1c ) can be evaluated from . The formation of easy domains may be accompanied with formation of a-domains normal to the a s2 -axis (hard domains), if, simultaneously with equation (8), the same condition is met for them, that is, Where . This is possible if (See Supplementary Equation 29 ). Thus, equation (10) is the necessary condition for the formation of a cross-hatched domain pattern on cooling from the cubic phase. If inequality in equation (10) is violated, stripe pattern forms. Moreover, the thickness dependence in equation (10) implies a qualitative conclusion: the formation of stripe patterns is more favourable for thicker films. In case of a c-monovariant, hard domain formation becomes favourable below T 2F (where ). However, the interaction of already existing easy domains with the appearing hard domains is associated with excess energy, impeding the formation of latter. Thus, the stripe pattern may persist through T 2F . On further cooling below T 2F , a cross-hatched pattern may or may not form, depending on the interplay between the two aforementioned factors. Further insight into this issue can be provided through phase-field simulations. The effect of anisotropy of the substrate on the transitions from 2-domain to 3-domain structures in similar systems has been previously studied [29] . Here, we are modelling the behaviour of the crossing between two narrow a-domain inclusions in order to investigate the interaction of the a-domains. The phase field simulation (see Methods) results in Fig. 1d–g (animated in Supplementary Movie ) illustrate the meta-stability of a-domain crossing. Small variation of simulation parameters like temperature, film thickness or domain wall energy (used in the presented case) decides whether the a-domain crossing is stabilized or not. Phase field calculated energies of distinct domain structures show that for realistic parameters at room temperature, three domain configurations: (i) c-mono-domain, (ii) periodic patterns of easy domains and (iii) cross-hatched pattern of a-domains, represent local energy minima. The structure with easy domains is the most stable. Wall pinning effect Domain wall pinning impedes the system from reaching the energy minimum, leading to domain patterns that deviate from the predictions of equilibrium theory. At equilibrium, film parameters are controlled by the coherency factor γ , which is temperature dependent. Ideally, during cooling from the paraelectric phase to the temperature of the experiment T exp , domain walls move to reach their equilibrium positions. Wall pinning interferes with this motion resulting that at T exp , γ takes a value γ * corresponding to a higher temperature. For typical temperature dependences of film and substrate lattice constants ( Fig. 1c ), γ increases with decreasing temperature, implying γ* < γ ( T exp ). In parallel, the a-domain width, w d , is an increasing function of γ , whereas the pattern period, l , is a decreasing one. Thus, wall pinning should lead to smaller w d and larger l compared with the equilibrium state. The theory above is introduced in terms of tetragonal system, but—in general—it can be adopted for other systems, for example, rhombohedral or orthorhombic. The key reason for the narrow domain formation in tetragonal film arises from the different mismatches of c- and a-domains with the substrate. The c-domain has almost zero mismatch, whereas both a-domains have above 4%. Analogical situation can be found, for example, in (111) oriented rhombohedral or (110) oriented orthorhombic systems. Both these systems have one ferroelastic state with out-of-plane elongation, which is the analogy to the c-domain, and several states with in-plane elongation, analogical to the a-domains. The theory can be adopted to any system where one domain state has a small mismatch with the substrate and another domain state a much larger mismatch of opposite sign. Making arrays of 10 nm wide domains We grew (see Methods) PZT (Zr:Ti=10:90) (001) tetragonal films, 50–230 nm thick, onto orthorhombic (pseudo-cubic) DyScO 3 (DSO) substrates whose weakly anisotropic in-plane lattice constants have a small positive mismatch with respect to the a-lattice constant of the PZT film. The topography evidences a highly controlled film growth and the ferroelectricity of the films was verified by hysteresis loop measurements (see Supplementary Figs 8 and 9 , respectively). From our theory, the selected substrate, exhibiting a weak anisotropy of in-plane lattice constants, is favourable for controlled formation of parallel stripe patterns of narrow a-domains. Although a strong anisotropy favours the formation of such patterns ( cf . equation (10)), it may prevent good film epitaxy. At the same time, for a weak anisotropy, stripe pattern is favoured by increasing film thickness (equation 10). The films were investigated by piezoresponse force microscopy (PFM; see Methods). The thinnest films (~50 nm) had a typical cross-hatched structure, in which the lines parallel to the [ ] S direction of the orthorhombic substrate were elongated (subscript s denotes the substrate), very often passing throughout the examined area, whereas the lines oriented along the substrate’s [001] S direction were much shorter and often broken by the former lines ( Fig. 2a ). Both small area PFM with a higher resolution (not shown) and transmission electron microscopy (TEM) cross-section images ( Fig. 2b ) reveal that the lines are very narrow a-domains, hence each dark line in Fig. 2a represents one a-domain and two domain walls. This is further emphasized by the high-resolution scanning TEM (HRSTEM) image in Fig. 2c . 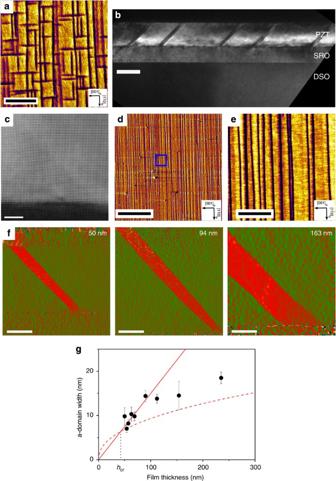Figure 2: Domain patterns and domain width in PZT films grown on DSO substrate. (a) 50 nm thick film: out-of-plane PFM amplitude map with yellow areas showing the piezoelectric activity of the c-domains and dark lines showing piezoelectrically inactive strips. The scale bar is 1 μm. (b) TEM and (c) HRSTEM cross-section of the film shown inaconfirming that the inactive strips ofaare a-domains. The scale bars are 50 and 5 nm, respectively. (d) 60 nm thick film: large-scale PFM scan showing a continuous parallel domain pattern throughout the whole scan range. Scan on different positions on the sample also show a purely parallel a-domain pattern parallel to the []Sdirection. The scale bar is 10 μm. (e) Magnification of the framed area ind, the scale bar is 1 μm. (f) Geometric phase analysis of HRSTEM images similar tocvisualizing the evolution of the a-domain width with the film thickness. The scale bar is 10 nm for the 163nm thick film and 20 nm for the others. (g) Measured width of a-domains in stripe domain patterns as a function of film thickness (data points). Theoretical prediction for the thickness dependence of the a-domain width in sparse a-domain patterns, equation (11), calculated using the lattice parameters of free standing PZT, obtained by analysis of the actual lattice parameters of our films (solid line). The minimum domain width predicted by the theory and evaluated using the material parameters of a PZT film taken from ref.1(dashed line). The crossing point marked withhcrcorresponds to the critical thickness for the domain formation given by equation (4). Figure 2: Domain patterns and domain width in PZT films grown on DSO substrate. ( a ) 50 nm thick film: out-of-plane PFM amplitude map with yellow areas showing the piezoelectric activity of the c-domains and dark lines showing piezoelectrically inactive strips. The scale bar is 1 μm. ( b ) TEM and ( c ) HRSTEM cross-section of the film shown in a confirming that the inactive strips of a are a-domains. The scale bars are 50 and 5 nm, respectively. ( d ) 60 nm thick film: large-scale PFM scan showing a continuous parallel domain pattern throughout the whole scan range. Scan on different positions on the sample also show a purely parallel a-domain pattern parallel to the [ ] S direction. The scale bar is 10 μm. ( e ) Magnification of the framed area in d , the scale bar is 1 μm. ( f ) Geometric phase analysis of HRSTEM images similar to c visualizing the evolution of the a-domain width with the film thickness. The scale bar is 10 nm for the 163nm thick film and 20 nm for the others. ( g ) Measured width of a-domains in stripe domain patterns as a function of film thickness (data points). Theoretical prediction for the thickness dependence of the a-domain width in sparse a-domain patterns, equation (11), calculated using the lattice parameters of free standing PZT, obtained by analysis of the actual lattice parameters of our films (solid line). The minimum domain width predicted by the theory and evaluated using the material parameters of a PZT film taken from ref. 1 (dashed line). The crossing point marked with h cr corresponds to the critical thickness for the domain formation given by equation (4). Full size image A transition to a purely parallel pattern was achieved by increasing the film thickness. This transition is observed at a critical thickness of about 60 nm. Films with thickness ~60 nm showed a-domains parallel to the [ ] S direction, whereas the domains in the [001] S direction disappeared completely ( Fig. 2d,e ). Often, the a-domains were continuous for tens of micrometres having the same orientation throughout the sample. The a-domains were very thin, typical domain width was ~10 nm for films of ~60 nm thickness. The width of the a-domains increased upon increase of the thickness of the film ( Fig. 2f,g ). Orientation of the miscut angle of the substrate did not influence the pattern ( Supplementary Fig. 10 ). The change of the pattern’s dimensionality upon increase of film thickness ( Fig. 2a versus 2d ) concurs with equation (10). To recall, this effect arises from the thickness dependence of the impact of the anisotropy on the formation energy of a-domains. The a-domain width, w d ( Fig. 2g ), shows a sub-linear dependence on the film thickness, h , which is actually linear at smaller thicknesses. This corroborates with our theoretical prediction of linear w d , versus h dependence in sparse a-domain patterns, equation (2). Using 0.3 for the Poisson ratio, equation (2) reads where ; at room temperature in DSO a s1 =0.39505, nm and a s2 =0.39468, nm. Equation (11) requires the use of the actual lattice constants of the film (in a free standing form), which often differ from the standard lattice parameters of the bulk material [31] . Taking this into account ( Supplementary Fig. 11 , derived using Supplementary Equations 41–46 ), we plot the solid line in Fig. 2g , showing the theoretical domain width for our case. In parallel, as we showed in equations (2) and (4), the domain width is bounded by the minimal possible value with h 0 =0.3 nm (ref. 1 ; the dashed line in Fig. 2g ). The crossing point of dependences given by equations (11) and (12) corresponds to the critical thickness for the domain formation given by equation (4). We also recall that domain wall pinning results in a smaller visible coherency factor γ , leading to a smaller domain width than the equilibrium one (area below the solid line in Fig. 2g ). Thus, our data points that deviate from the linear law (equation 11) suggest pinning effects in the thicker films. Repair of misbehaving domain-arrays Although our theory does not predict any ‘thick’ regime, films having thickness beyond 100 nm exhibited often cross-hatched a-domain pattern ( Fig. 3a , right). However, as it was mentioned in the theoretical part of the paper, the stipe pattern on further cooling may become cross-hatched, explaining such pattern in the thickest films. Alternatively, the structure of the thicker films might originate from defect and dislocation issues. To further elucidate this, a set of three films having different domain patterns in as-grown state ( Fig. 3a ) were subjected to thermal treatment: after heating to 550 °C and a short stabilization period of 5 min, they were cooled to room temperature at 1.5 °C min −1 (tenfold slower than post-growth cooling rate). The domain pattern is depicted in Fig. 3b . Following this, the films were soaked again at the same 550 °C and cooled down with 15 °C min −1 (same rate as after growth), resulting in the domain pattern shown in Fig. 3c . 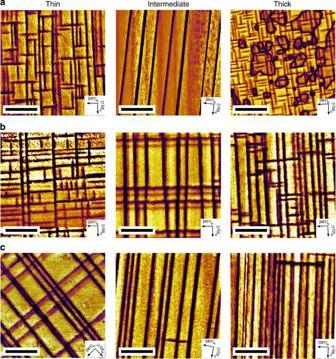Figure 3: Effect of annealing on domain structure. Out-of-plane PFM amplitude of thin (<60 nm), intermediate (>60 nm) and thick (>100 nm) films (a) in the as-grown state, (b) after thermally cycling and slow cooling and (c) after an additional thermal cycle and fast cooling. The size of the scale bar is 1 μm. Figure 3: Effect of annealing on domain structure. Out-of-plane PFM amplitude of thin (<60 nm), intermediate (>60 nm) and thick (>100 nm) films ( a ) in the as-grown state, ( b ) after thermally cycling and slow cooling and ( c ) after an additional thermal cycle and fast cooling. The size of the scale bar is 1 μm. Full size image The domain pattern of the thick films transformed to now become strikingly similar to the ‘intermediate thickness’ films. This suggests that the high density of defects is reduced, as they can heal at elevated temperature. The lowered defect density allows the theoretically predicted anisotropic domain pattern to form. This suggests that the random domain structure, often reported in literature, is likely to be signature of high defect density. For the intermediate-thickness films, the slow cooling resulted in appearance of cross-hatched patterns. However, these patterns did not resemble those of the thin films. Instead of exhibiting short a-domains confined by the perpendicular ones, mostly a-domain crossings can be observed. A fast cooling of the films allowed recovery of the previously existing long-range parallel domain pattern ( Fig. 3c , centre). The possibility to reversibly modify the domain pattern between a parallel and a cross-hatched pattern adds a further route for domain-structure control. In contrast, the thin films remained cross-hatched also under fast cooling, the thickness being too low to violate condition (10) for the given lattice parameter anisotropy of the substrate. Towards complex patterns As is known, domain walls often display properties different from those in the bulk and we may expect, for example, their elevated conduction. However, there exists a strong reason that particularly the ultrathin a-domains—and their domain walls—between mismatched c-domains may display additional strong deviation of functional properties compared with larger domains in differently strained films. Although the c-domain regions are almost unstrained, the a-domains have >4% mismatch with the substrate. In fact, this mismatch is the reason for small a-domain width. The a-domains are therefore exposed to several competing forces. First, large in-plane compressive stress is applied to the a-domain close to the substrate because of their mismatch. Second, an a-domain is exposed to the tensile stress from neighbouring c-domains. Third, the elastic mismatch between a- and c- domains is suppressed by the flat substrate resulting in a sheer stress in and around the a-domains. Combined, the appearance of an a-domain induces large inhomogeneous strains, which may be described as local strain engineering. Obviously, the local stresses must affect also the domain walls, which, as seen from our simulation and TEM data and also seen by others [32] , are bent off the ideally electrically neutral and elastically compatible flat parallel orientations. It is appealing therefore to create more complex ordered patterns. 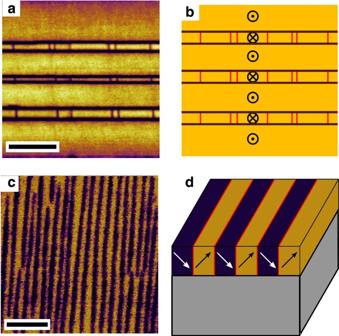Figure 4: Domain configurations obtained by post-growth writing onto during-growth controlled domain patterns. (a) PFM micrograph of domain pattern obtained by post-growth writing of c-domains onto PZT films with stripe a-domain arrays. The scale bar is 1 μm. (b) Schematic drawing of the pattern shown ina,⊙depicts c-domain with polarization up,⊗c-domain with polarization down, red vertical lines a-domains, brown horizontal lines 180° domain walls. (c) One-dimensional dense domain array (here domain width ~20 nm) in PZT film grown with an originally monovariant domain structure on (110) SrTiO3substrate and manipulated through post-growth switching with PFM tip moving perpendicular to the direction of the formed domain stripes. The scale bar is 200 nm. (d) Schematic drawing of the pattern shown inc, the arrows indicate the direction of the polarization. Figure 4a,b shows the combination of as-grown fine ferroelectric/ferroelastic domain stripes superimposed with post-growth PFM-written purely ferroelectric (180°) walls. With expected differences in properties of 180° walls and properties of ultrafine a-domains, such a structure could potentially make an electronic circuit. In contrast to the sparse patterns shown above, a 20-nm wide dense domain stripes are shown in Fig. 5c,d . Such patterns, reminiscence of those observed in BiFeO 3 (ref. 33 ), were obtained in monodomain 60-nm thick PZT films grown on (110) SrTiO 3 substrate and post-growth switched with the PFM tip moving perpendicular to the direction of the so-formed domain stripes. Figure 4: Domain configurations obtained by post-growth writing onto during-growth controlled domain patterns. ( a ) PFM micrograph of domain pattern obtained by post-growth writing of c-domains onto PZT films with stripe a-domain arrays. The scale bar is 1 μm. ( b ) Schematic drawing of the pattern shown in a , ⊙ depicts c-domain with polarization up, ⊗ c-domain with polarization down, red vertical lines a-domains, brown horizontal lines 180° domain walls. ( c ) One-dimensional dense domain array (here domain width ~20 nm) in PZT film grown with an originally monovariant domain structure on (110) SrTiO 3 substrate and manipulated through post-growth switching with PFM tip moving perpendicular to the direction of the formed domain stripes. The scale bar is 200 nm. ( d ) Schematic drawing of the pattern shown in c , the arrows indicate the direction of the polarization. 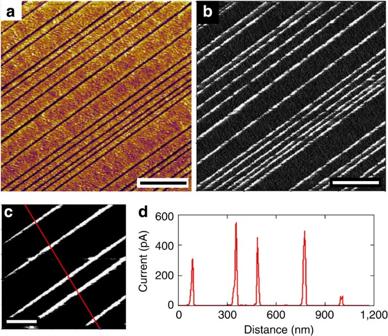Figure 5: Conductivity of a-domains. (a) PFM amplitude image measured on 60 nm film with stripe domain pattern immediately after (b) c-AFM map measured with sample bias of +4.5 V. The scale bar is 1 μm. (c) Small area c-AFM map measured under same conditions, scale bar is 250 nm. (d) Current versus distance plotted along the red line crossing the c-AFM map inc. Full size image Figure 5: Conductivity of a-domains. ( a ) PFM amplitude image measured on 60 nm film with stripe domain pattern immediately after ( b ) c-AFM map measured with sample bias of +4.5 V. The scale bar is 1 μm. ( c ) Small area c-AFM map measured under same conditions, scale bar is 250 nm. ( d ) Current versus distance plotted along the red line crossing the c-AFM map in c . Full size image Electrical properties of the stripe domain arrays We measured the electronic properties of the ultrafine a-domains by Conductive Atomic Force Microscopy (c-AFM). The domain pattern remained unchanged after the conduction measurements, as confirmed by PFM images ( Fig. 5a ) taken before and after c-AFM scans. The conduction map measured on a 60-nm thick film with stripe domain pattern ( Fig. 5b ) closely reproduces this pattern, where robust conduction (up to 600 pA in comparison with the<0.2 pA of the rest of the film) clearly marks the position of the narrow a-domains. Conduction in PZT was reported only for artificially created 180° domain walls [34] , where a transport mechanism based on defect-mediated hopping enhanced by defect segregation at domain walls was proposed. Such a mechanism could be applicable also for the case studied here. To gain a deeper insight, a 1 × 1 μm 2 map was taken ( Fig. 5c ). The conduction peak width at half maximum is 15–25 nm ( Fig. 5d ), which is close to the a-domain width. Similar (or wider) peak width is typically measured on a single-domain wall, for example, in ref. 34 . Hence, whether the observed current peaks represent overlapping conductive traces of two domain walls or of the entire a-domains requires further detailed investigation. Of importance is that the stripe arrays of narrow a-domains exhibited unexpected robust and potentially useful conductive properties. We developed phenomenological theory showing ways to obtain stripe arrays of ultrathin ferroelastic/ferroelectric domains. Using phase-field models, we tested the sensitivity of various configurations to indicate stability of the domain structures under different conditions. Based on this, we elaborated films of classical PZT, showing consistently stripe arrays of 10 nm wide a-domains inside c-domain matrix. We showed a possibility to modify ‘wrong’ domain patterns by post-growth thermal treatment. The narrow a-domains were conductive in contrast to the insulating matrix. In view of the degree of control of the fine patterns and the demonstrated conductivity, and considering previous reports on unique electronic and magnetic properties of ferroelectric domain walls, it is appealing to envision future electronic circuits based on tailored domain walls and domain patterns. Sample preparation Thin PbZr 0.10 Ti 0.90 O 3 (PZT) and SrRuO 3 (SRO) films were grown by pulsed laser deposition from a self-made target onto (110) DSO substrates with a miscut angle of 0.1° (CrysTec GmbH) towards the [ ] S direction. The laser had a wavelength of 248 nm and the energy density used was 1 J cm −2 . During the SRO bottom layer growth, the substrate was kept at T S =625 °C in an oxygen pressure p O2 =0.145 mbar. To deposit the PZT layer, T S =575 °C and p O2 =0.25 mbar were used. Subsequent to deposition, the films were cooled down at 15 °C min −1 and p O2 =1 mbar. At room temperature, the a axis of the PZT ( a =0.3914, nm, c =0.4138, nm) [35] has a mismatch of 0.93% and 0.84% in the [001] S and [ ] S directions of the (110) DSO (0.39505 and 0.39468, nm) [36] , respectively. At deposition temperature, the lattice parameter of PZT as derived by Landau theory [18] , [37] is 0.4009, nm giving an average misfit of −0.35%. This small compressive mismatch allows for the growth of coherent films of high quality. As can be seen from TEM ( Fig. 2b ), the obtained PZT layer is monocrystalline, exhibiting no grain-boundaries or other extended defects. Lattice mismatch between PZT and substrate causes strain contrast inside the PZT layer close to the interface. Additional strain arises at the tips of the a-domains, extending into the SrRuO 3 bottom electrode. TEM TEM was done with a Philips CM300 instrument (Philips) using an acceleration voltage of 300 kV. The HRSTEM experiments were performed on an FEI Titan 50–300 PICO microscope at an operating voltage of 200 kV. Geometric phase analysis [38] is used to process the high-angle annular-dark-field images. PFM The PFM was performed using an Asylum Research Cypher AFM (Asylum Research). For the c-AFM, measurements were carried out using the same AFM system with an Asylum ORCA current preamplifier. Conductive Asylec Ti/Ir-coated probes with nominal force constant 3 N m −1 were used for all c-AFM scans presented in this paper. Sample bias of +4.5 V was used. Note that for this bias polarity the out-of-plane polarization component does not switch. Same probes were used for PFM measurements in order to verify that the domain pattern remained unchanged after the c-AFM scan. The phase-field model The results of phase-field model ( Fig. 1a,d–g ) were obtained by the numerical solution of three-dimensional versions of the time-dependent Landau–Ginzburg–Devonshire equation, Poisson’s equation for dielectrics and equation of motion in elastic material as described in Supplementary Materials of ref. 6 . Here the equations are solved under the condition of zero defect concentration, zero free carrier concentration, with material parameters corresponding to PZT (Zr:Ti=10:90) from ref. 37 , and with gradient energy terms G 11 =4.14 × 10 −10 Jm 3 C −2 , G 12 =0 Jm 3 C −2 and G 44 =2.07 × 10 −10 Jm 3 C −2 . In the model geometry, the block of (001) oriented PZT film with thickness from 15 to 50 nm ( Fig. 1a shows the case of 30 nm) is mechanically coupled with a block of (110) S DSO substrate, which is three times thicker and governed only by equation of motion as purely elastic material. The elastic stiffness of DSO is assumed identical to that of cubic PZT. The lattice mismatch between PZT and DSO and the substrate orthorhombic distortion are introduced by setting an artificial in-plane spontaneous strain to DSO. The film and substrate have defined periodic boundary conditions (with 150 nm period) in x and y directions. The PZT surfaces perpendicular to the z-direction have zero electric potential representing fully screened surface polarization charge. The block of PZT is mechanically free (has zero out-of-plane stress) on upper surface and the substrate bottom surface has clamped mechanical displacement in z -direction ( z axis points ‘up’). The initial conditions of polarization are set as shown in Fig. 1a where the polarization modulus has bulk spontaneous value at room temperature. Initial electric potential in the film is zero and the initial mechanical displacement corresponds to stress-free substrate in the whole model. The model is numerically solved by the finite element method with a time-dependent solver in COMSOL 4.3a until stationary solution is reached. Variations of simulation parameters, including initial conditions (with two, one or no a-domains), temperature, film thickness and domain wall energy, were tested to indicate stability of the domain structure. How to cite this article: Feigl, L. et al . Controlled stripes of ultrafine ferroelectric domains. Nat. Commun. 5:4677 doi: 10.1038/ncomms5677 (2014).